Model-based rational design of an oncolytic virus with improved therapeutic potential Oncolytic viruses are complex biological agents that interact at multiple levels with both tumour and normal tissues. Antiviral pathways induced by interferon are known to have a critical role in determining tumour cell sensitivity and normal cell resistance to infection with oncolytic viruses. Here we pursue a synthetic biology approach to identify methods that enhance antitumour activity of oncolytic viruses through suppression of interferon signalling. On the basis of the mathematical analysis of multiple strategies, we hypothesize that a positive feedback loop, established by virus-mediated expression of a soluble interferon-binding decoy receptor, increases tumour cytotoxicity without compromising normal cells. Oncolytic rhabdoviruses engineered to express a secreted interferon antagonist have improved oncolytic potential in cellular cancer models, and display improved therapeutic potential in tumour-bearing mice. Our results demonstrate the potential of this methodology in evaluating potential caveats of viral immune-evasion strategies and improving the design oncolytic viruses. Oncolytic viruses (OVs) are promising anticancer therapeutics engineered or selected to infect and multiply specifically in tumour cells while having attenuated replication capacity in normal tissues [1] , [2] . The attenuation of OV growth in normal tissues is often due to the inability of OVs to antagonize normal cellular, interferon (IFN)-mediated antiviral responses. Many tumour cells have acquired defects in their IFN response during their malignant evolution, and are correspondingly excellent hosts for OV growth [3] , [4] , [5] , [6] , [7] . However, the extent of the IFN response deficit in cancers is highly variable and can impair the efficacy of OV therapies [8] . This has led to intensive efforts aiming at suppressing IFN signalling in tumour cells without compromising the antiviral programmes in normal tissues [9] , [10] . Although previous mathematical models have been developed to describe the kinetics of OV replication [11] , [12] , [13] , [14] , the field of OV engineering has yet to adopt approaches from Synthetic Biology, where mathematical models are often used to guide the development of biological systems. To demonstrate the potential of model-based rational design of OVs, we combined mathematical modelling and viral genome engineering to design and test strategies that might allow evasion of the IFN response in the tumour microenvironment, while maintaining safety in normal tissues. Whether a patient receives therapeutic virus intravenously [15] or through direct intratumoural injection [16] , the quantity of virus that reaches the tumour bed is vastly outnumbered by the number of target cells found in the malignancy [17] . Successful OV therapies thus rely upon the ability of a relatively small number of virus particles to initiate an infection and spread within a population of cancer cells. Viruses are strictly dependent upon the biosynthetic machinery of the infected host cell to produce progeny particles. Correspondingly, cancer cells that are rapidly dividing and have established robust biosynthetic machinery inherently produce larger numbers of virus particles when compared with cells in normal tissue, which are quiescent and have a restricted ability to synthesize new nucleic acids and proteins [18] , [19] . In cancer cells, this effect is exasperated by defects in immune responses, which further enhance viral replication. In a simple model of virus infection, the distinction between viral replication kinetics in healthy and tumour tissue is characterized by differences in available biosynthetic machinery and innate immune responses ( Fig. 1 ). When virus is delivered to normal tissue, it infects a limited number of cells creating a subpopulation, producing both virus progeny and IFN. As the infection proceeds, slow virus replication enables the IFN-mediated defence response to outpace virus particle production and restrict infection. Viruses that can prevent the production of IFN from infected cells, or stimulate host cell metabolism, are correspondingly expected to have an increased capacity to spread within normal tissues. Indeed pathogenic viruses incorporate both these strategies into their life cycle [20] , [21] . In tumours non-responsive to the antiviral effects of IFN, invading virus will co-opt the biosynthetic machinery of the cancer cell producing large numbers of virus particles. In this setting, the virus will rapidly spread and destroy the malignancy. In tumours responsive to IFN, virus spread will be favoured by the high metabolic rate of the cancer, but at the same time limited by the ability of neighbouring cells to mount an innate immune antiviral response. In this setting, it is the balance between virus production and the extent of initiation of antiviral responses that will ultimately determine the therapeutic outcome. 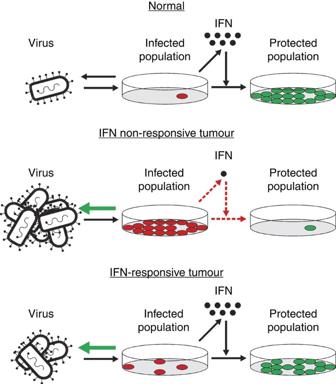Figure 1:Model development. Comparison of virus replication dynamics in three tissue types: normal cells, IFN non-responsive tumours and IFN-responsive tumours. Processes enhanced relative to normal cells are illustrated in green, whereas those impaired are illustrated in red. Figure 1: Model development . Comparison of virus replication dynamics in three tissue types: normal cells, IFN non-responsive tumours and IFN-responsive tumours. Processes enhanced relative to normal cells are illustrated in green, whereas those impaired are illustrated in red. Full size image Model simulations of different IFN-evading strategies To simulate virus infection and spread within tumour and normal tissue, we developed a phenomenological model describing the varied ability of different cell types to support virus proliferation. In this model, cells within an ‘uninfected population’ transitions into an ‘infected population’ (IP) upon viral infection. The number of infected cells in the IP increases over time, as virus is produced and spreads to neighbouring cells. Production of IFN from IP cells allows these cells to transition into an ‘activated population’ (AP) where viral defenses slow virus release and further enhance IFN production. Over time, this population will gradually become a ‘protected population’ (PP) of cells that have cleared the infection and maintain active antiviral defense programmes [22] , [23] , [24] . We used this phenomenological model as the basis for simulating the outcome of different IFN-evasion strategies on three types of cells: normal cells, IFN non-responsive tumour cells and IFN-responsive tumour cells. We assumed that these cell types differ mainly in their ability to facilitate virus replication and to activate IFN. By quantifying cytotoxicity induced 72 h post infection in each of these three cell types, the simulations seek to explore how the relationship between virus replication, activation of IFN-mediated defense responses and cytotoxicity induced across the population might be exploited to design improved therapeutic strategies. Because of the heterogeneity of tumour and healthy cells, and the corresponding uncertainty associated with kinetic parameter estimates, we further employed a Monte Carlo sampling method to simulate 1E4 different combinations of kinetic parameters randomly sampled within one order of magnitude from values reported in the literature. The outcome of this unbiased method are probability distributions describing the susceptibility of each of the three simulated types of cells towards viral infection. We first asked if the model could recapitulate the effects associated with an attenuating mutation in the natural wild type (WT) isolate of vesicular stomatitis virus (VSV), (wild type (WT)), which renders the virus sensitive to IFN signalling, here referred to as Δ51 (ref. 6 ). In VSV WT, functional M-protein blocks IFN production to enable viral evasion of the immune response [25] . As expected, VSV WT is highly efficient in infecting and killing both normal and tumour populations ( Fig. 2a ). In agreement with experimental observations in a variety of tumour models [6] , [26] , [27] , our simulations predict that the Δ51-attenuated virus will eradicate IFN non-responsive tumours, whereas normal populations or IFN-responsive tumours will be largely resistant ( Fig. 2c ). 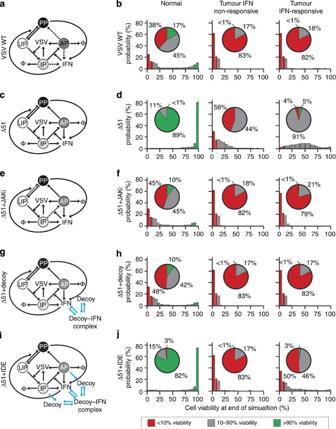Figure 2: Simulation of IFN-evasion strategies on rhabdovirus-induced cytotoxicity. The phenomenological model was amended to describe treatment with (a) VSV WT, (c) Δ51, (e) Δ51 in the presence of a JAKi, (g) Δ51 in the presence of a DR for IFN and (i) Δ51-mediated expression of the IFN DR (Δ51-IDE). Colour coding highlights processes impaired (dashed) or gained (blue) relative to Δ51. Each of the above models used a Monte Carlo sampling method to generate the probability distribution of population viability following treatment with (b) VSV WT, (d) Δ51, (f) Δ51+JAKi (h), Δ51+decoy (j) Δ51-IDE for 72 h in normal cells (left) and tumours with non-responsive (tumour IFN-NR; centre) or responsive (tumour IFN-R; right) IFN signalling pathways. Colour coding, quantified in pie charts, describes the probability that each of the three cell types has a viability <10% (red), 10–90% (grey) or >90% (green) at the end of the simulation. Figure 2: Simulation of IFN-evasion strategies on rhabdovirus-induced cytotoxicity. The phenomenological model was amended to describe treatment with ( a ) VSV WT, ( c ) Δ51, ( e ) Δ51 in the presence of a JAKi, ( g ) Δ51 in the presence of a DR for IFN and ( i ) Δ51-mediated expression of the IFN DR (Δ51-IDE). Colour coding highlights processes impaired (dashed) or gained (blue) relative to Δ51. Each of the above models used a Monte Carlo sampling method to generate the probability distribution of population viability following treatment with ( b ) VSV WT, ( d ) Δ51, ( f ) Δ51+JAKi ( h ), Δ51+decoy ( j ) Δ51-IDE for 72 h in normal cells (left) and tumours with non-responsive (tumour IFN-NR; centre) or responsive (tumour IFN-R; right) IFN signalling pathways. Colour coding, quantified in pie charts, describes the probability that each of the three cell types has a viability <10% (red), 10–90% (grey) or >90% (green) at the end of the simulation. Full size image We next tested two scenarios to determine whether chemical manipulation of the IFN responses of virus-infected cell could enhance the activity of Δ51 in IFN-responsive tumours, while maintaining a low impact in normal populations. Simulations of Δ51 infection in the presence of a chemical inhibitor that blocks IFN signalling (for example, a JAK inhibitor (JAKi)) predict a toxicity profile reminiscent of infection with VSV WT ( Fig. 2e ). Although the inhibition of IFN signalling increases virus effectiveness against tumours, it also causes the normal population to become highly susceptible to infection. This outcome is also predicted to occur in simulations where the population is exposed to a biological agent that prevents IFN interaction with its cognate receptor (for example, a soluble IFN receptor antagonist; Fig. 2g ). We then tested the idea of coupling the production and secretion of the decoy receptor (DR) to virus replication. In this model, Δ51 is engineered to synthesize a soluble IFN-binding DR only when viral gene expression is initiated, thereby creating a positive feedback loop. Positive feedback sharpens dose responses and enables all-or-none switching in cellular signalling pathways [28] , and might thus drive specificity towards the tumour environment. The results obtained by simulating the cytotoxicity induced upon infection with the Δ51 IFN decoy-expressing (IDE) virus (Δ51 IDE ) were highly encouraging ( Fig. 2i ). Specifically, the simulated efficacy towards tumours was significantly increased compared with the unmodified Δ51 virus, without posing additional risk of damage to the normal population even at high doses of the virus ( Supplementary Fig. S1 ). Experimental testing of simulation predictions in vitro To test the model predictions, we performed experiments to compare the efficacy and specificity of Δ51 under each of the simulated IFN-evasion strategies. We previously identified the renal carcinoma cell line 786-0 as having a partially intact IFN response and being refractory to killing by Δ51 (refs 9 , 29 ). Correspondingly, experiments were performed by the cotreatment of IFN-responsive tumour cells (786-0) and normal fibroblast (MRC5) cells with the Δ51-GFP virus in the presence of the JAKi or exogenously added recombinant B19R-soluble IFN DR [30] , [31] , [32] , [33] , [34] . In agreement with the outcome predicted by our simulations, the presence of the chemical inhibitor increased Δ51-mediated killing of 786-0 tumour cells, but equally resulted in a loss of specificity as MRC5 normal cells became susceptible to infection ( Fig. 3a ). Similar results were obtained when the two cell types were cultured in the presence of the DR protein before Δ51 treatment ( Fig. 3a and Supplementary Fig. S2 ). 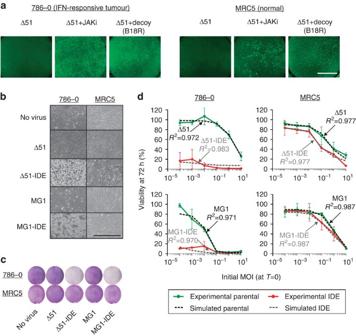Figure 3:Validation of model predictionsin vitro. (a) Infection of resistant tumours with functional IFN defenses (786-0) and normal (MRC5) cells with Δ51-GFP at a multiplicity of infection of 0.1 in the presence or absence of 10 μM of the JAKi or 0.1 μg ml−1of the B19R DR. Microscopy images were taken 48 h post infection. Scale bar, 2 mm in length. (b) Cytopathic effects of the Δ51-IDE as observed by bright-field microscopy 24 h post infection. Scale bar, 500 μm in length. (c) Cytopathic effects of the Δ51-IDE as observed by crystal violet staining 72 h post infection. Images are from a 12-well plates (2.5 cm diameter). (d) Experimental and simulated relationship between multiplicity of infection and cellular viability 72 h post infection. Error bars represent the s.d. from triplicate technical replicates. Trends represent the simulation, which best describes the experimental results. Figure 3: Validation of model predictions in vitro . ( a ) Infection of resistant tumours with functional IFN defenses (786-0) and normal (MRC5) cells with Δ51-GFP at a multiplicity of infection of 0.1 in the presence or absence of 10 μM of the JAKi or 0.1 μg ml −1 of the B19R DR. Microscopy images were taken 48 h post infection. Scale bar, 2 mm in length. ( b ) Cytopathic effects of the Δ51-IDE as observed by bright-field microscopy 24 h post infection. Scale bar, 500 μm in length. ( c ) Cytopathic effects of the Δ51-IDE as observed by crystal violet staining 72 h post infection. Images are from a 12-well plates (2.5 cm diameter). ( d ) Experimental and simulated relationship between multiplicity of infection and cellular viability 72 h post infection. Error bars represent the s.d. from triplicate technical replicates. Trends represent the simulation, which best describes the experimental results. Full size image To test the prediction that virus performance can be improved by incorporating an IFN-suppressing positive feedback loop, we incorporated the B19R IFN DR into the Δ51 backbone, and a second IFN-sensitive attenuated OV derived from the Maraba virus termed MG1 ( Supplementary Fig. S3 ). This second rhabdovirus was used to evaluate the generality of the strategy, and because MG1 is a more aggressive rhabdovirus with more potent oncolytic activity as compared with Δ51 (ref. 35 ). We refer to these IDE viruses as Δ51 IDE and MG1 IDE , respectively. After confirming the expression and activity of the DR produced from these viruses ( Supplementary Fig. S3 ), we performed a microarray analysis of differential genome-wide transcription upon infection. This analysis confirmed that IFN decoy expression following viral infection leads to a significant repression of the type I IFN response in IFN-producing cells ( Supplementary Fig. S4 and Supplementary Table S1 and Supplementary Data 1 and 2 ). As predicted by our simulations, both Δ51 IDE and MG1 IDE viruses were associated with tumour-selective cytotoxicity. In the 786-0 tumour cell line, both strains were associated with a greater cytopathic effect than their attenuated parental virus strains. However, neither of the IDE viruses caused significant damage to MRC5 normal cell ( Fig. 3b ). We next examined the effect of varying initial virus concentrations on cell viability using both our computer model and cell culture experimentation. Remarkably, we were able to achieve excellent quantitative agreement between the model simulations and experimental data in the above cell lines ( Fig. 3d ), or in alternative models ( Supplementary Fig. S5 ). To establish whether spreading between the cancerous and normal cell compartments compromises safety, we performed a series of coculture experiments. To first assess if IDE viruses have increased spreading ability, we deposited virions in the centre of a monolayer of 786-0 cells and examined cell death caused by virus spreading 48 h post infection ( Fig. 4a ). Both Δ51 IDE and MG1 IDE viruses were superior to their parental counterparts in terms of their ability to rapidly spread through a 786-0 monolayer. Quantification of the surface area affected revealed that virus penetrance was increased sevenfold for Δ51 IDE and fourfold for MG1 IDE ( Fig. 4b ). Similar results were obtained using alternative tumour cell lines and methods ( Supplementary Fig. S6 ). In contrast, IDE viruses had no detectable spread in normal GM38 cells. We next performed our coculture spreading assay by adding pre-infected 786-0 cells onto a monolayer of normal fibroblasts, and monitored viability 72 h post infection by crystal violet staining. Parental WT viruses (VSV WT or Maraba) spread from the infected tumour cells into surrounding normal cell culture causing widespread off-target killing ( Fig. 4c ). On the other hand, Δ51/MG1 were restricted only to the local tumour microenvironment and had their spreading rapidly blunted by the normal cell monolayer. Finally, the Δ51 IDE and MG1 IDE viruses were indistinguishable from their attenuated parental counterparts, and lacked the ability to spread into a normal cell monolayer, suggesting that the engineered IFN-suppressing positive feedback loop does not compromise normal tissue ( Fig. 4c ). 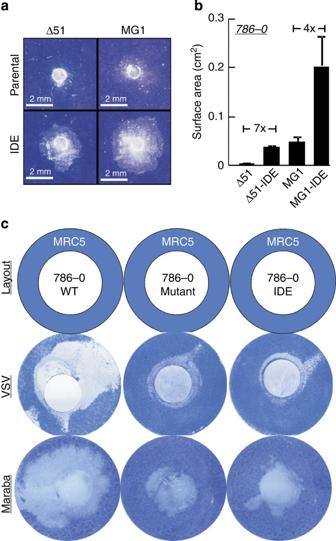Figure 4: Viral spreading. (a) Comparison of virus spreading by crystal violet staining in 786-0 cells. Scale bar, 2 mm in length. (b) Quantification of virus spreading surface. Error bars represent the s.d. from triplicate technical replicates. (c) Coverslip spreading assay. The 786-0 cells were plated in a dish containing round coverslip and infected at a multiplicity of infection of three during 4 h. The round coverslip was transferred on a monolayer of naive MRC5 cells and an agarose overlay was added on the top. Five days later, cells were fixed and stained with Coomassie brilliant blue. Images are from a six-well plates (3.5 cm diameter). Figure 4: Viral spreading. ( a ) Comparison of virus spreading by crystal violet staining in 786-0 cells. Scale bar, 2 mm in length. ( b ) Quantification of virus spreading surface. Error bars represent the s.d. from triplicate technical replicates. ( c ) Coverslip spreading assay. The 786-0 cells were plated in a dish containing round coverslip and infected at a multiplicity of infection of three during 4 h. The round coverslip was transferred on a monolayer of naive MRC5 cells and an agarose overlay was added on the top. Five days later, cells were fixed and stained with Coomassie brilliant blue. Images are from a six-well plates (3.5 cm diameter). Full size image Efficacy and specificity of IDE viruses in vivo To test the in vivo activity of the IDE viruses, we established subcutaneous tumours in BALB/c mice using an IFN-responsive variant of the murine CT26 colon tumour cell line. In our initial studies, animals were treated with OVs intravenously and were killed at various times to quantitate the level of virus replication in normal and tumour tissues ( Fig. 5a ). Consistent with earlier studies [6] , virus was cleared from normal organs whether or not it expressed an IFN decoy by day 4. However, the Δ51 IDE and MG1 IDE viruses persisted longer and grew to higher titres in the tumour tissue than in their parental counterparts. 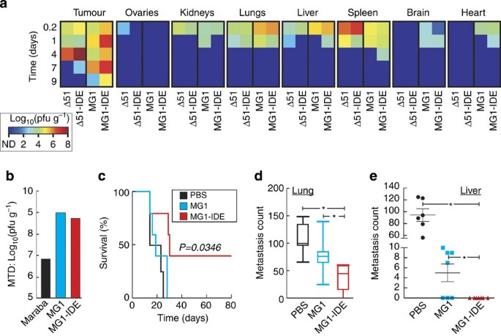Figure 5:Safety and efficiency of a decoy-expressing virusin vivo. (a) Biodistribution in CT26 tumour-bearing BALB/c mice injected with 1E8 pfu i.v. (b) maximum tolerated dose in tumour-naive BALB/c mice. (c) Survival study of immunodeficient mice bearing an HT29 subcutaneous tumour treated with 1E8 pfu injected i.v. (n=5). (d) CT26 tumour cell metastasis to the lung in BALB/c mice following treatment with 1E7 pfu injected i.v. (n=7). Box plot illustrates the sample maximum and minimum (error bars), Q1 and Q3 (box), and the median of the population (central bar). (e) CT26 tumour metastasis to the liver in BALB/c mice following treatment with 1E8 pfu injected i.v. (PBS,N=6; MG1s,N=7). *Statistical difference between groups (one-way analysis of variance,P<0.0001; two-tailed heteroscedastict-test,P<0.05). Figure 5: Safety and efficiency of a decoy-expressing virus in vivo . ( a ) Biodistribution in CT26 tumour-bearing BALB/c mice injected with 1E8 pfu i.v. ( b ) maximum tolerated dose in tumour-naive BALB/c mice. ( c ) Survival study of immunodeficient mice bearing an HT29 subcutaneous tumour treated with 1E8 pfu injected i.v. ( n =5). ( d ) CT26 tumour cell metastasis to the lung in BALB/c mice following treatment with 1E7 pfu injected i.v. ( n =7). Box plot illustrates the sample maximum and minimum (error bars), Q1 and Q3 (box), and the median of the population (central bar). ( e ) CT26 tumour metastasis to the liver in BALB/c mice following treatment with 1E8 pfu injected i.v. (PBS, N =6; MG1s, N =7). *Statistical difference between groups (one-way analysis of variance, P <0.0001; two-tailed heteroscedastic t -test, P <0.05). Full size image We also tested the efficacy of MG1 IDE in a number of tumour settings after confirming that the maximum tolerated dose was minimally affected by addition of the DR ( Fig. 5b ). In a human xenograft model using the HT29 cell line, MG1 IDE clearly outperformed its parental MG1 strain, effecting long-term cures in ∼ 50% of the animals ( Fig. 5c and Supplementary Fig. S7 ). We next established CT26–LacZ colon tumours in the lungs of BALB/c mice by intravenous (i.v.) infusion to assess the impact of IDE on metastatic tumour clearance ( Fig. 5d ). Mice were injected with CT26–LacZ i.v. and 3 days later with 1e7 pfu of virus. Mice were killed 13 days after cell injection. CT26 metastases were counted and results clearly show an increase in efficacy associated with the IDE virus. This result could be further improved in a liver metastasis model in immunocompetent mice where 100% of the mice treated with MG1 IDE were liver tumour free ( Fig. 5e ). Taken together, these results indicate that IDE rhabdoviruses improve the therapeutic potential of OVs without compromising toxicity in normal tissue. OVs are advancing through late-phase randomized clinical trials, and it seems likely that one or more products will be approved in the near future [36] , [37] , [38] , [39] , [40] . Despite encouraging clinical data, it is clear that the genetic heterogeneity of tumours will make it necessary to create novel OVs to maximize their potential as anticancer agents. Here, we evaluated whether model-based rational design could be used to design OVs. After implementing the model to characterize various prevalidated attenuating strategies, such as the Δ51 mutation [6] or engineering VSV WT to express IFN ( Supplementary Fig. S8 ) [41] , we sought to predict novel methods that would increase tumour killing in IFN-responsive tumours without compromising normal tissues. Our model simulations demonstrated that an indirect positive feedback loop, generated through virus-mediated expression of a DR, should selectively enhance virus-mediated cytotoxicity within the tumour microenvironment in excellent agreement with subsequent experimental observations. These simulations provide the theoretical framework describing the advantages of incorporating a DR into the backbone of OVs. By allowing a DR to be encoded by the virus, the functional impact of the repressor on virus kinetics is delayed, as its expression requires the establishment of a productive viral infection. Repressor-mediated enhancement of viral replication can only occur in the environment surrounding cells predisposed towards viral infection and replication. When virus particles enter adjacent normal tissue where viral replication is slow or aborted, levels of the DR should be gradually lost, thereby preventing the systematic spread of the virus in normal tissue. By using a synthetic biology approach to rationally designed OVs, we have established a methodology that allows the potential caveats of various immune-evasion strategies to be evaluated. This method has allowed us to identify those with the greatest probability of success, and has resulted in the development of two novel oncolytic candidates. Biological materials and reagents Vesicular stomatitis viruses are as follows: Δ51 (ref. 6 ), Δ51-GFP, VSV WT and Δ51 IDE . Maraba Spanish double-mutant virus MG1 and MG1 IDE were both generated by Stojdl and colleagues [35] . The following cell lines used were obtained from the American Type Culture Collection (Manassas, VA): African Green Monkey kidney (Vero), human renal cancer cells (786-0), murine colon cancer cells (CT26), human colon cancer cells (HT29), mouse melanoma cancer cells (B16), human glioma cancer cells (U251), primary human fibroblast cells (GM38) and human (MRC5). All cells were grown in DMEM (Hyclone Laboratories Inc.) with 10% FBS (Invitrogen, Burlington, ON, Canada). Recombinant B19R (VACWR200) utilized in this study was obtained from eBioscience, Inc. (San Diego, CA), and the JAKi was purchased from EMD Millipore. Construct validation For the cloning, mRNA expression of the IFN–DR expression from new rhabdoviruses constructs was verified by PCR. For primers used, see Supplementary Table S2 . For the microarray analysis, RNA extraction was performed 24 h post infection in 786-0 cells. Duplicate samples were pooled and hybridized on Affymetrix human gene 1.0 ST arrays according to manufacturer instructions. Data analysis was performed using AltAnalyze [42] . Briefly, probeset filtering implemented a DABG threshold of 70 with P <0.05 and utilized constitutively expressed exons. Genes differentially expressed were identified using a combination of a >1.5-fold change in expression and a significance of P <0.05 (Student’s t -test) ( Supplementary Data 1 ). Gene ontology enrichments were performed using GOrilla [43] ( Supplementary Data 2 ). Identification of genes induced by type I IFNs was performed using the interferome database [44] . For both cloning and microarray analysis, RNA was collected using an RNeasy kit (Qiagen, Toronto, Ontario, Canada). In vitro analysis For in vitro cell death and cytopathic effects assays, cell lines were plated in 12-well plates at 3E6 cells per well. Twenty-four hours later, cells were treated with each of the five different regimens. Seventy-two hours post infection, crystal violet (0.1%) staining was performed to visualize live cells. Bright-field images were taken with a Zeiss Axiovert S100 Inverted Microscope. For the Alamar Blue Assay, 5E4 cells were plated in 96-well plates. After 24 h, cells were infected with each virus. Forty-eight hours post infection, 10 μl of the Alamar blue reagent (Invitrogen) was added to each well. Reading was done using the Labsystems Fluoroskan II Fluorescent Microplate Reader using the Em/Ex 590/530 nm filters. For spreading assays, cells were plated in six-well plates at 8E5 cells per well. After 24 h, the cells were covered with a 0.7% agarose overlay containing antibiotics (Penicillin and Streptomycin) in which a small hole was made in the middle of the well where 5E3 pfu of virus was injected. After 5–6 days incubation, crystal violet staining or VSV immunostaining assessed virus spread. VSV antibodies (polyclonal antibodies from immunized mouse) targeting whole virus were utilized at a dilution of 1/800 and left for a duration of 30 min before being washed off with water. For coverslip spreading assays, MRC5 cells were plated into a 10-cm-well dish until 100% confluence was obtained after 24 h. The 786-0 cells were plated in a six-well plates containing a sterile coverslip at a density to reach 100% confluence after 24 h. The 786-0 cells were then infected at an multiplicity of infection of five for 4 h. Coverslips were removed and placed on the dish containing MRC5 cells and were covered by a 0.5% agarose/2 × DMEM overlay. Five days later, virus spreading was assayed by crystal violet staining. Animal experiments All animal experiments were performed in accordance with institutional guidelines review board for animal care (John C Bell and University of Ottawa ethical board). For safety study, biodistribution assay was performed by injecting 3E5 CT26–LacZ cells subcutaneously on the right side of a BALB/c mouse. Seven days later, tumours were administered 1e8 pfu of each virus intravenously (i.v.). Organs titred and collected 0.2, 1, 4, 7 and 9 days post infection include the brain, lungs, ovaries, spleen, liver, kidneys, heart and tumour. The maximum tolerated dose assay was performed using a dose escalation of Maraba, MG1 and MG1IDE between 5E8 and 5E9 pfu administered i.v., and monitoring the dose keeping 100% of mice alive. For efficacy testing in the HT29 model, 3E6 cells were injected subcutaneously in nude mice. Seven days post tumour embedding, mice were treated with PBS, MG1 or MG1IDE at 1E8 pfu administered i.v. In the CT26–LacZ model, 1E5 CT26–LacZ cells were injected via the tail vein into BALB/c mice. Mice were treated with MG1 and MG1IDE (1e7 pfu) i.v. on day 3. Thirteen days post tumour implantation, mice were killed and the lungs were excised and stained with X-gal solution before counting. In the liver metastases model, 1E6 CT26–LacZ cells were administered intrasplenic into BALB/c mice using intrasplenic/portal injection. Four days after, 1E8 pfu of virus was injected i.v. as treatment. Fourteen days after tumour cell injection, mice were killed and the spleen/liver were collected and stained with X-Gal before counting. Modelling Our model describing OV replication dynamics ( Supplementary Fig. S9 ) is represented by a subset of eight ordinary differential equations. The first four equations describe the transition between the uninfected population, IP, AP and PP depending on the concentration of virus and IFN in the environment. These equations are as follows: The parameters used in the above equations represent the infection rate ( K VI ), the rate of IFN signalling activation ( ), the rate of IFN signalling inactivation ( ), the EC50 of IFN (EC50), the rate of cell death ( ) and the rate viral clearance ( ). The next subset of equation describe the concentration of virus (V), IFN, DR and DR–IFN complex in the media. These equations are as follows: The parameters described in the above equations represent the rate of virus budding from IP and AP ( and , respectively), the infection rate ( K VI ), the rate of virus degradation ( ), the rate of IFN production from IP, AP and PP ( , and , respectively), the rate of IFN degradation ( ), the rate of DR production from IP and PP ( and , respectively), the rate of decoy degradation ( ), the forward rate of IFN–DR complex formation ( ) and the reverse rate of complex formation ( ). IFN-responsive tumours were simulated by decreasing and tenfold relative to normal cells. IFN non-responsive tumours were simulated equally by randomly decreasing all IFN-regulated processes ( , , , and ) 2- to 20-fold. The Monte Carlo simulation was generated by varying the parameters in the above model within a 1-log window. Model parameter identification was performed using a simulated annealing method where all parameters are identical in a given cell line other than the capacity to produce IDE. All simulations were generated in Matlab using the ODE solver ode15s under default parameters, imposing a none-negativity constraint. A full list of model amendments to describe each IFN-evasion strategy, as well as a list of parameter values utilized in our simulations, are available in Supplementary Tables S3 and S4 , respectively. Accession codes : Microarray data has been deposited in Array Express under accession code E-MTAB-1636 . How to cite this article: Le Bœuf, F. et al . Model-based rational design of an oncolytic virus with improved therapeutic potential. Nat. Commun. 4:1974 doi: 10.1038/ncomms2974 (2013).